Crackling noise in fractional percolation Crackling noise is a common feature in many systems that are pushed slowly, the most familiar instance of which is the sound made by a sheet of paper when crumpled. In percolation and regular aggregation, clusters of any size merge until a giant component dominates the entire system. Here we establish ‘fractional percolation’, in which the coalescence of clusters that substantially differ in size is systematically suppressed. We identify and study percolation models that exhibit multiple jumps in the order parameter where the position and magnitude of the jumps are randomly distributed—characteristic of crackling noise. This enables us to express crackling noise as a result of the simple concept of fractional percolation. In particular, the framework allows us to link percolation with phenomena exhibiting non-self-averaging and power law fluctuations such as Barkhausen noise in ferromagnets. Many systems crackle when pushed slowly. Examples include the crumpling of paper [1] , earthquakes [2] , solar flares [3] , the dynamics of superconductors [4] and the magnetization of slowly magnetized magnets. For a piece of wood in fire one can even hear crackling noise without special equipment. Across all systems that display crackling noise, the order parameter of the system exhibits randomly distributed jumps, and discrete, spontaneous events span a broad range of sizes [5] . Magnification of the hysteresis curve of a magnetic material in a changing external field, for instance, reveals that the magnetization curve is not smooth but exhibits small discontinuities. This series of correlated jumps is called the Barkhausen effect, which is a standard example for crackling noise in physics [6] , [7] , [8] . Despite its importance, crackling noise is far from being understood. In random network percolation a fixed number of nodes are chosen randomly, and two of them are connected according to certain rules [9] , [10] , [11] , [12] . This procedure is repeated over and over again until every node is connected to every other. Once the number of added links exceeds a certain critical value, extensively large connected components (clusters) emerge that dominate the system. The reverse process is called fragmentation, see Fig. 1 . Fragmentation processes, where homogeneous parts break up into smaller ones, are ubiquitous and have been studied intensely. The applications range from disintegration of atomic nuclei, and the fragmentation of glass rods, to fracture in large-scale systems [13] , [14] , [15] , [16] , [17] , [18] , [19] . An important observation is that the size of the fragments are of the same order of magnitude as the parent pieces. Thus, the case where one fragment is microscopic while the size of the other fragment is substantially larger is rare. 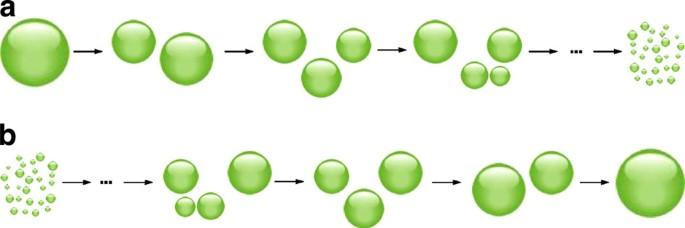Figure 1: Fragmentation and fractional percolation. (a) In the process of fragmentation, clusters split up into parts of a certain fraction. (b) The reverse dynamics, ‘fractional percolation’, is studied here. In contrast to ordinary aggregation processes, in fractional percolation the coalescence of clusters that substantially differ in size is systematically suppressed. Figure 1: Fragmentation and fractional percolation. ( a ) In the process of fragmentation, clusters split up into parts of a certain fraction. ( b ) The reverse dynamics, ‘fractional percolation’, is studied here. In contrast to ordinary aggregation processes, in fractional percolation the coalescence of clusters that substantially differ in size is systematically suppressed. Full size image Here we model this by systematically suppressing asymmetric break ups. This suppression suggests a fractional increase of clusters, that is time-reversed fragmentation. We demonstrate that crackling noise in percolation unexpectedly emerges from this simple fractional growth rule. To further demonstrate the universality of our approach, computer simulations for the proposed percolation mechanism in geometrical confinement are carried out. The particular model we use to exemplify the fractional growth mechanism can be replaced by any other model where first a fixed number of nodes are chosen at random, and then two nodes are connected, according to any rule that forbids the largest chosen component to merge with components smaller than a fixed fraction of its size. As we will reveal by a single event analysis, the network model features three basic properties: (i) a fractional growth mechanism, (ii) a threshold mechanism and (iii) a mechanism that amplifies critical fluctuations. We show that these underlying mechanisms account for the main features of crackling noise. Perhaps most importantly, the framework allows us to derive macroscopic features from the underlying micro-dynamical mechanisms, which exposes connections between the seemingly unrelated concepts of percolation, fragmentation and crackling noise. Network model Consider a network with a fixed number of nodes N and L links. Start with N isolated nodes and no links, L =0. At each step, choose three different nodes v 1 , v 2 and v 3 uniformly at random. Let S 1 , S 2 and S 3 denote the sizes of the (not necessarily distinct) clusters they reside in. Assume S 1 ≥ S 2 ≥ S 3 , and 0< f ≤1 is fixed. Connect those two nodes v i and v j for which Δ ij := fS i − S j , 1≤ i < j ≤3 is minimal, see Fig. 2 . If necessary, choose randomly among multiple minima, whose corresponding nodes are to be linked. Hence, a certain type of size homophily among clusters is applied, where connections between two clusters are preferred, which are similar in size, after the size of the larger cluster has been rescaled by a factor f , the ‘target fraction’. As Δ 12 ≤Δ 13 , only Δ 12 and Δ 23 have to be considered. The rule is also applied if the nodes to be linked reside in the same component. As a ‘final rule’, when there are only two clusters left in the system, connect these. For single realizations of the process, see Fig. 3 . As seen in the study, fragmentation as S →( gS := S i , (1− g ) S := S j ) with is the inverse process, and the target fraction f determines the magnitude of the discontinuities in the order parameter. 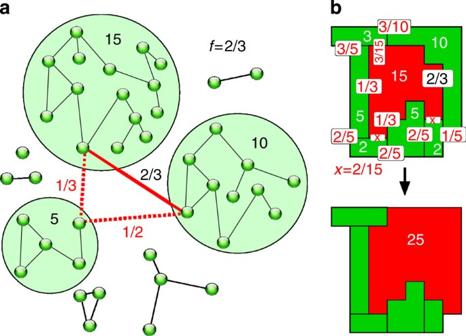Figure 2: Sketch of the models. (a) Select three nodes at random and calculate the sizes of the clusters they reside inS1≥S2≥S3. Connect those two nodesνiandνj, which reside in clusters that minimize Δij:=fSi−Sjamong Δ12, Δ13and Δ23, where 0<f≤1 is fixed. (Actually, it is unnecessary to consider Δ13as Δ12≤Δ13). Here a link between the clusters of size 15 and 10 is established because the (arbitrarily chosen) fixed target fractionf=2/3 is here exactly met: Δ12=2/3 × 15−10=0<Δ23=2/3 × 10−5=5/3<Δ13=2/3 × 15−5=5. (b) Lattice model. Draw randomly a focal cluster (red) and merge those two neighbour clusters that minimize Δ (see text). Figure 2: Sketch of the models. ( a ) Select three nodes at random and calculate the sizes of the clusters they reside in S 1 ≥ S 2 ≥ S 3 . Connect those two nodes ν i and ν j , which reside in clusters that minimize Δ ij := fS i − S j among Δ 12 , Δ 13 and Δ 23 , where 0< f ≤1 is fixed. (Actually, it is unnecessary to consider Δ 13 as Δ 12 ≤Δ 13 ). Here a link between the clusters of size 15 and 10 is established because the (arbitrarily chosen) fixed target fraction f =2/3 is here exactly met: Δ 12 =2/3 × 15−10=0<Δ 23 =2/3 × 10−5=5/3<Δ 13 =2/3 × 15−5=5. ( b ) Lattice model. Draw randomly a focal cluster (red) and merge those two neighbour clusters that minimize Δ (see text). 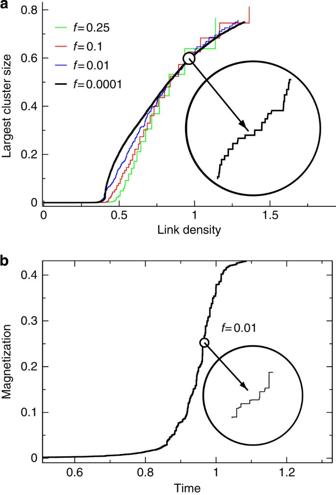Figure 3: Discontinuous jumps. (a) Scheme of crackling noise in network percolation. Single realizations of fractional percolation processes for the network sizeN=218. The evolution of the largest componentS1/Nis displayed. The control parameterfdetermines the magnitude of the discontinuities. In the thermodynamic limitN→∞, the process shows infinitely many discontinuous jumps. (b) Same for the magnetization of the Barkhausen model on a square lattice,N=400 × 400, single realization forf=0.01. Full size image Figure 3: Discontinuous jumps. ( a ) Scheme of crackling noise in network percolation. Single realizations of fractional percolation processes for the network size N =2 18 . The evolution of the largest component S 1 / N is displayed. The control parameter f determines the magnitude of the discontinuities. In the thermodynamic limit N →∞, the process shows infinitely many discontinuous jumps. ( b ) Same for the magnetization of the Barkhausen model on a square lattice, N =400 × 400, single realization for f =0.01. Full size image Let us order the largest components of the system by S 1 , S 2 , …, with sizes s 1 = S 1 / N ≥ s 2 = S 2 / N …, and write ‘with high probability’ (whp) to express that the probability of a certain statement gets arbitrarily close to 1 as N →∞. The link density of the network is the analogue of the occupation probability for lattices and defined by p = L / N , where L denotes the number of links that have been added to the network. Let p c characterize the critical link density, the position of the (first) phase transition. We show next that an arbitrarily fractional increase of components features discontinuities that survive even in the thermodynamic limit, and that this implies non-self-averaging [15] . Self-averaging A thermodynamic quantity, such as the total magnetization or the size of the largest component in a networked system s 1 , is self-averaging if its relative variance becomes zero in the thermodynamic limit [15] , where the brackets denote ensemble averaging. For non-self-averaging systems, however, the thermodynamic quantity remains broadly distributed for large systems and large sample sizes. Systems that lack self-averaging therefore lack the collapse of the ensemble average, and its minimum and maximum as well. Non-self-averaging has an important role in the statistical physics of disordered systems, for instance in spin glasses [15] , [20] , [21] , neural networks, polymers and population biology [22] , [23] . We characterize non-self-averaging in percolation [24] , [25] by a non-vanishing relative variance of the order parameter s 1 on an extended interval. For investigating this, it is helpful to study the underlying microscopic mechanisms in terms of a single event analysis. Fractional growth mechanism First we show that, for f >0, the largest component cannot merge with components smaller than . If less than three distinct clusters are picked, either an intracluster link is added and the size of largest component is necessarily unchanged, or the size of the largest component doubles. Thus, we consider the case of three distinctly chosen components whose sizes are ordered, ≥ ≥ . Proof by contradiction: Assume Δ 1,2 is minimal such that and merge when (A) . In fact, Δ 1,3 is never minimal (except if it is equal to another Δ) as Δ 1,3 ≥Δ 1,2 , and if Δ 2,3 was minimal then the largest chosen cluster would not merge with any other. By multiplying A with f and adding − we obtain . As Δ 1,2 is minimal, we have f − < f − , and hence we obtain f , which is impossible for f >0. Thus, either stays constant, increases ‘fractionally’ by at least a factor of or is overtaken (by a merger of and ). However, overtaking becomes unlikely as the size of the largest component increases. Impossibility of ( N ) overtaking By ( N ) overtaking, we mean the merger of two components, each smaller than the largest component, which together are larger than the largest component and of size ( N ). Our line of arguments holds for any rule based on picking at most three nodes randomly. Assume that S 1 = ( N ), considering the following cases. Case (i): Both smaller components are ( N ). This is (whp) impossible because the upper limit for the number of macroscopic components is 2. Actually for any n -node rule (where first n nodes are chosen randomly followed by any other rule), there cannot exist more than n −1 macroscopic clusters over any extended period of time [26] . Case (ii): At least one of the smaller components is o ( N ). In this case, overtaking is (whp) impossible as either S 1 ≥ S 2 ′+ S 3 ′ or S 1 → S 1 + o ( N ). Threshold mechanism Taken together, for the infinite system, this implies that as soon as the size of the second largest component exceeds , the second largest component merges with the largest one, s 1 → s 1 + s 2 . As a third macroscopic component is (whp) impossible, this also implies the reset of the second largest component, s 2 →0. Power law fluctuations by amplification of critical fluctuations Summarizing the above considerations, after the first-phase transition, for p > p c and N →∞, the size of the largest component either stays constant or jumps discontinuously. As the first transition is point-continuous [24] , [27] , [28] , the process necessarily exhibits infinitely many discontinuous transitions arbitrarily close to the first transition point, p = p c . Let δ n denote the height of the n th step down the staircase. The fractional growth mechanism suggests the proportionality δ n ~ g n , where . This yields the jump size distribution for f >0, where δ (·) denotes the Delta function and γ is a constant. This is supported by numerics (see Fig. 4 ). 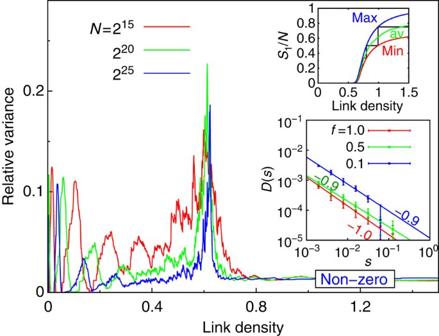Figure 4: Non-self-averaging crackling noise in the network model. The relative varianceof the largest component in dependence on the link densitypis displayed,f=1. Forp>pcthe system is non-self-averaging characterized by→const.>0, forN→∞. Upper inset: Stochasticity of transition points characterized by the lack of the collapse of average, minimum and maximum values ofS1, here shown forf=1 and an ensemble of 500 realizations. A single realization is displayed in black. Lower inset: As derived in the text, for anyf>0,N→∞, the jump sizes are power law distributed,D(s)~s−τ(τ=1 theory). Fit exponentsτf=1=0.96±0.06 (R=0.990),τf=0.5=0.85±0.03 (R=0.998) andτf=0.1=0.90±0.04 (R=0.997). Error bars indicate standard deviations. Figure 4: Non-self-averaging crackling noise in the network model. The relative variance of the largest component in dependence on the link density p is displayed, f =1. For p > p c the system is non-self-averaging characterized by →const.>0, for N →∞. Upper inset: Stochasticity of transition points characterized by the lack of the collapse of average, minimum and maximum values of S 1 , here shown for f =1 and an ensemble of 500 realizations. A single realization is displayed in black. Lower inset: As derived in the text, for any f >0, N →∞, the jump sizes are power law distributed, D ( s )~ s − τ ( τ =1 theory). Fit exponents τ f =1 =0.96±0.06 ( R =0.990), τ f =0.5 =0.85±0.03 ( R =0.998) and τ f =0.1 =0.90±0.04 ( R =0.997). Error bars indicate standard deviations. Full size image The stochasticity is a consequence of the exponential amplification of the critical fluctuations of s 1 at the first-phase transition point, p c . Fluctuations, measured by the relative variance, in the size of the largest component s 1 at p c are known to be non-zero, ( s 1 ( p c ))>0 (refs 9 , 27 ). From δ n ≈ εg n , we see that uncertainties ε are exponentially suppressed as n increases. In contrast, fluctuations in s 1 at p c are exponentially amplified, for increasing p . As a result, both the size of the jumps, and the transition points are stochastic—even for the infinite system. Thus, the process is non-self-averaging, characterized by a non-vanishing relative variance This is numerically supported, see Fig. 4 , and stands in contrast to the weakly discontinuous case (see Supplementary Methods and Supplementary Figs S1–S3 ). Expressing δ n in terms of a time-dependent target fraction f ( n ), and assuming f ( n )= α / n , 0< α ≤1, from equation (2), we obtain D ( s )~ characterizing power law fluctuations that decay faster than ~ s −1 . Thus, other fluctuation types than ~ s −1 are accessible via a non-constant f . Barkhausen percolation model As clusters in our framework neither have a magnetization nor are geometrically confined, the analogy to magnetic effects such as the Barkhausen effect, a standard example of crackling noise in geometrical confinement, remains incomplete. To demonstrate the universality of our claims, next we study a Barkhausen percolation model on a square lattice. Assume that each cluster has a homogeneous magnetization; either m ( S i )=0 or m ( S i )=1. Initially all sites are single clusters and have m =0, up to a set of sites of o ( N ) that is set to m =1, for example, a few single clusters. Now apply repeatedly the following update rule. (i) Uniformly draw a cluster at random, (ii) among this focal cluster and its (von Neumann-) neighbours, merge those two neighbour clusters that minimize Δ:= fS i − S j (see Fig. 2b ), (iii) magnetization: apply the neutral rules 0+0→0, and 1+1→1, together with the magnetization rule 0+1→1, for the merging clusters. In addition, apply the physical time increment rule t → t +min( s i , s j ) 1/2 at each merger, s i and s j being the scaled cluster sizes of two merging components. This rule accounts for cracks preceding a fragmentation. Cracks have a finite propagation velocity, which implies that duration of a fragmentation event depends on the size of the fragments [15] , [29] . Here we have arbitrarily chosen the square root of the smaller cluster as the time increment. However, the main features of the model are independent of the specific choice. Fragmentation mimics the repeated reconfiguration of homogeneous magnetic domains under a slowly increased opposite external magnetic field. A magnetic domain is a region within a ferromagnetic material with uniform magnetization. During the demagnetization, domains split up into smaller ones of different magnetization, a process called reconfiguration. This is in most ferromagnetic materials the dominating factor in the minimization of the local magnetostatic energy and accounts for the sudden jumps of the total magnetization in the hysteresis curve. However, due to other effects, the process stops when the domain size approaches a threshold, usually in range of 10 −4 to 10 −6 m (refs 5 , 8 ). Here we demonstrate that the reverse process, fractional percolation, reproduces the main features of Barkhausen noise. While only a caricature of the intricate processes in ferromagnets [6] , [7] , it nonetheless explains multiple randomly distributed discontinuous jumps in the total magnetization , together with non-SA, and power law fluctuations, see Fig. 5 , Supplementary Methods and Supplementary Figs S4–S7 . 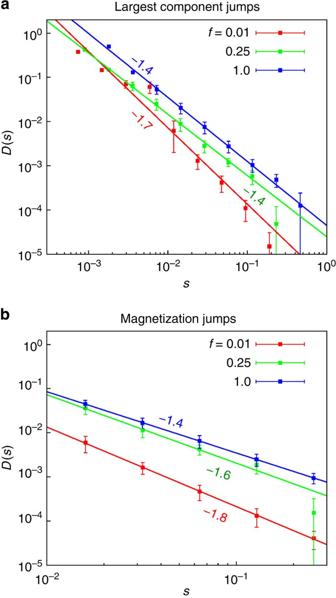Figure 5: Power law fluctuations in the lattice model. Power law fluctuations (a) in the largest cluster size, and (b) in the total magnetization. The jump size distributionsD(s)~s−τsuggest a power law decay. Lattice sizeN=500 × 500 (periodic boundary conditions). Initial condition with a single magnetized cluster. Jumps smaller than the relative size 7 × 10−4are discarded. Data points are averaged over 1,000 realizations, using logarithmic binning. Distributions without using log-bins are shown inSupplementary Fig. S6. Error bars indicate standard deviations. (a) Fit exponentsτf=0.01=1.7±0.2 (R=0.983),τf=0.25=1.4±0.03 (R=0.999) andτf=1=1.4±0.04 (R=0.999). (b) Fit exponentsτf=0.01=1.8±0.02 (R=0.999),τf=0.25=1.6±0.07 (R=1.00) andτf=1=1.4±0.01 (R=1.00). Figure 5: Power law fluctuations in the lattice model. Power law fluctuations ( a ) in the largest cluster size, and ( b ) in the total magnetization. The jump size distributions D ( s )~ s − τ suggest a power law decay. Lattice size N =500 × 500 (periodic boundary conditions). Initial condition with a single magnetized cluster. Jumps smaller than the relative size 7 × 10 −4 are discarded. Data points are averaged over 1,000 realizations, using logarithmic binning. Distributions without using log-bins are shown in Supplementary Fig. S6 . Error bars indicate standard deviations. ( a ) Fit exponents τ f =0.01 =1.7±0.2 ( R =0.983), τ f =0.25 =1.4±0.03 ( R =0.999) and τ f =1 =1.4±0.04 ( R =0.999). ( b ) Fit exponents τ f =0.01 =1.8±0.02 ( R =0.999), τ f =0.25 =1.6±0.07 ( R =1.00) and τ f =1 =1.4±0.01 ( R =1.00). Full size image We have established crackling noise in percolation. In particular, we have demonstrated analytically that fractional growth rules imply randomly distributed jumps in the order parameter. These jumps are discontinuous phase transitions. However, when such mechanisms are mixed, even weakly, with mechanisms that merge components purely at random then the transitions vanish, or become at most weakly discontinuous characterized by very small power law exponents [30] , [31] , [32] , [33] , [34] , [35] , [36] , [37] , [38] , [39] , [40] , [41] , see Supplementary Methods and Supplementary Figs S1–S3 . Fractional percolation describes nucleation where domains cannot grow in arbitrarily small pace. As an application consider an unmagnetized ferromagnetic sample of linear dimension of about l =1 cm at room temperature. It is not unrealistic to assume that the magnetic domains have roughly the same linear dimension l 0 =10 −3 cm, independent of l , but different magnetizations that globally compensate each other. An increasing external magnetic field typically causes magnetic domains to increase at least by the size of one of its neighbour domains. Thus, this mechanism alone would result in the total magnetization to either stay constant or jump in steps of the size of magnetic domains. As long as l 0 >0, this quantized growth is an example of the fractional growth rule as the largest domain cannot increase by arbitrarily small amounts. However, as we increase the sample size, the ratio l 0 / l decreases such that for the infinite system any jump size becomes zero relative to the system size. Thus our framework suggests that Barkhausen noise is at most ‘weakly discontinuous’. In fact, in many soft magnetic materials Barkhausen jump sizes are not extensive and thus their relative size shrinks with increasing system size [8] . In contrast, in thin magnetic films and other geometries where long-range interactions are not of major importance, macroscopic jumps have been reported [42] . The characteristics of fractional percolation are robust against an arbitrary (time-dependent) variation of the parameter f >0 that determines the magnitude of the discontinuities. The framework combines mechanisms reminiscent of many physical and biological systems: the order parameter exhibits a sudden jump upon exceeding a dynamical threshold [5] , [29] , [43] , [44] , and large-scale fluctuations emerge as a consequence of critical fluctuations. The amplification and propagation of critical fluctuations to macroscopic scales has been subject of intensive investigations in quantum critical systems, such as the inflationary expansion of the early universe [45] , and disordered systems exhibiting quenched disorder [20] , [21] . However, the current understanding of most systems where randomness is frozen or amplified is far from being complete. A recent study on group formation in small growing populations, for instance, shows that the fraction of one trait within the population (for example, cooperators) can be subject to strong fluctuations as a result of the amplification of stochastic fluctuations generated during the initial phase of the dynamics [46] , [47] . Power law fluctuations across operating scales, discontinuous jumps of the order parameter and non-self-averaging may considerably subvert predictability and control of networked systems [11] , [48] . Exact conditions for these phenomena are elusive [15] . Our analysis provides sufficient conditions for these features. Because the framework connects the seemingly unrelated concepts of percolation, fragmentation and crackling noise, it might help to qualitatively improve the understanding of systems that display (stochastic) discontinuous phase transitions. In short, we expressed the main features of crackling noise as a consequence of a simple concept: fractional percolation. Mixed model For a general argument, we introduce a stochastic mix of two processes, ordinary Erdös-Renyí (ER) percolation, and the simple model of fractional percolation introduced in the main text. Consider a graph G ( ν , ε ), where the vertex set ν has N nodes, and the edge set ε has L links. Start with N isolated nodes and an empty set of edges . With probability q , connect two randomly chosen different nodes (that is, ER rule), otherwise, at each step, choose three different nodes v 1 , v 2 and v 3 uniformly from V (for fractional percolation) and follow the steps given in the main text (choose the minimal Δ), see Supplementary Fig. S1 . Global continuity for q >0 Consider any rule based on picking a fixed number of nodes randomly, which is applied, at each step with probability 1− q , such as fractional percolation, or other types of discontinuous percolation, together with an ER-type process, which is applied with probability q , such as ER percolation. Here, by ER-type process, we mean a percolation process, based on randomly choosing a fixed number of nodes, which does not allow the emergence of more than a single giant component because it would instantaneously merge with any other macroscopic component of size ( N ). After the first-phase transition, that is, for p > p c a giant component necessarily must have emerged. Hence, for fixed q >0 and N →∞ there is no extended interval ( p c , p * > p c ) in which macroscopic components smaller than the largest one can emerge, because the ER-type rule would merge them infinitely often with the largest one in any extended subinterval. This cannot be compensated even by high rates of the creation of components of size ( N ), because at any given time there exist at most 1/ α components of size αN , or greater for α >0. As a result, for p > p c all components smaller than the largest one are at any time of o ( N ), and discontinuous jumps in s 1 are therefore impossible. Clearly, for p < p c all components S 1 , S 2 ,… are microscopic, that is of size o ( N ). As any rule based on randomly picking a fixed number of nodes is necessarily point-continuous at the first transition point p=p c (refs 24 , 25 ), the order parameter s 1 , the size of largest cluster, is globally continuous and we can state that, for q >0, the process is globally continuous. Barkhausen percolation model The size of the largest cluster necessarily displays a stochastic staircase on an extended interval after t c , where t c is the first-phase transition point, for N →∞. Large randomly distributed jumps of the total magnetization are a consequence of this. For the Barkhausen model on a square lattice (introduced in main text), numerical evidence is presented that the total magnetization exhibits discontinuous jumps, and displays power law fluctuations together with non-self-averaging. Single realizations of the Barkhausen model are shown in Supplementary Fig. S4 . In contrast to the self-averaging case shown in Supplementary Fig. S3 , Fig. S5 indicates that the relative variance of M (and S 1 ) is non-zero on a finite interval and does not shrink to a single peak for N →∞. In addition, Supplementary Fig. S6 provides numerical evidence for large-scale fluctuations, for all values of the parameter f . In ordinary square lattice percolation, the critical window (around the phase-transition point t c ) is characterized by fluctuations that decay as D ( s )~ s − τ , with τ ≈2.0. For the thermodynamical limit, the exponent is exactly known, τ =187/91 (ref. 9 ). For small values of f , an exponent close to τ =1.7 is observed here. In contrast, we find larger fluctuations exhibiting a decay closer to a power law with exponent 3/2, for f =0.25, and f =1. We expect this fluctuation type for finite systems with a sufficiently high tendency for the suppression of the growth of large clusters—in stark contrast to ordinary percolation. More precisely, the assumption that the cluster sizes develop similarly to percolation in 1d, or equivalently, to the ‘global competition model’ studied in Nagler et al . [31] , leads to the prediction , where T is the (unscaled) time, that is the number of added links or bonds, and n and T are connected via the identity (ref. 31 ). Finite size fluctuations in the critical window are then expected to follow , where the prime indicates the derivative. Hence, , for some constant γ >0. This result is in agreement with the numerical results shown in Supplementary Fig. S6 , for not too small values of f . In contrast, this behaviour is expected to vanish in the limit N →∞. In this limit, fractional percolation on a lattice is expected to exhibit D ( s )~ s −1 , as a consequence of the stochastic staircase on a finite interval (see main text). However, the studied system sizes do not allow to observe this behaviour with statistical significance, as the size of the critical window is too large for the studied system sizes, implying D ( s )~ s −3/2 . Nevertheless, the statistics of large fluctuations of the magnetization for f =1 is not inconsistent with D ( s )~ s −1 . For the lattice model, the fact that the stochastic staircase is extended after t c is a result of the physical time increment rule t → t +min( s i , s j ) (introduced in the main text). This particular rule accounts for the finiteness of the crack propagation velocity. Importantly, for t > t c any other size-dependent delay also leads to (i) discontinuous transitions that are (ii) randomly distributed (non-self-averaging) together with (iii) large-scale fluctuations. In agreement with the framework, for the studied system sizes, we numerically find the largest gap in M (and S 1 ) to be effectively independent of the system size, see Supplementary Fig. S7 . Therefore we have demonstrated strong numerical evidence that the Barkhausen process involves macroscopic broadly distributed jumps in the total magnetization, together with non-self-averaging. How to cite this article: Schröder, M. et al. Crackling noise in fractional percolation. Nat. Commun. 4:2222 doi: 10.1038/ncomms3222 (2013).